Ribosomal DNA copy number is coupled with gene expression variation and mitochondrial abundance in humans Ribosomes are essential intracellular machines composed of proteins and RNA molecules. The DNA sequences (rDNA) encoding ribosomal RNAs (rRNAs) are tandemly repeated and give origin to the nucleolus. Here we develop a computational method for estimating rDNA dosage (copy number) and mitochondrial DNA abundance using whole-genome short-read DNA sequencing. We estimate these attributes across hundreds of human genomes and their association with global gene expression. The analyses uncover abundant variation in rDNA dosage that is coupled with the expression of hundreds of functionally coherent gene sets. These include associations with genes coding for chromatin components that target the nucleolus, including CTCF and HP1β . Finally, the data show an inverse association between rDNA dosage and mitochondrial DNA abundance that is manifested across genotypes. Our findings uncover a novel and cryptic source of hypervariable genomic diversity with global regulatory consequences (ribosomal eQTL) in humans. The variation provides a mechanism for cellular homeostasis and for rapid and reversible adaptation. Copy number variation (CNV) is a significant source of natural genetic diversity. The ribosomal RNAs (rRNAs) are essential structural and catalytic components of ribosomes, are conserved throughout all domains of life and are encoded in repetitive loci (ribosomal DNA (rDNA) arrays) that might be among the most copy number (CN) hypervariable genomic segments. However, the functional consequences of rDNA CN polymorphisms are unknown and often assumed to be negligible. The eukaryotic ribosome is an indispensable cellular machine composed of a core complex of ~80 proteins and 4 rRNA molecules. The mature 80S ribosome consists of the small 40S (containing the 18S rRNA) and large 60S (containing the 28S, 5.8S and 5S rRNAs) subunits, each with distinct functions [1] . In humans, the 18S, 5.8S and 28S rRNA molecules are encoded within tandemly repeated 43-kb nucleolar organizing regions residing on the five acrocentric autosomal chromosomes (13, 14, 15, 21 and 22) [2] ( Fig. 1 ), while the 5S rRNA is encoded by a tandemly repeated ~2.2-kb cluster on chromosome 1 (1q42 region) [3] . In addition, ~150 proteins and ~70 small nucleolar RNAs interact or are associated with the ribosome during its biogenesis [4] . Remarkably, transcription from the rRNAs constitutes over 80% of cellular RNAs with thousands of ribosomal subunits synthesized each minute in actively growing eukaryotic cells [5] , [6] . Considering the pivotal role of the ribosome, it is of little surprise that a number of diseases are traced to defective ribosomal proteins and deficient rRNA transcription [7] . Mitochondria, the organelles responsible for energy production, are also critical for cellular function, contain their own genome (~16.5 Kb) independent from the nucleus ( Fig. 1 ), are present at variable levels in cells and interact with nuclear ribosomes through coordinated processes [8] , [9] , [10] . Indeed, functional relationships between the rRNA transcription and the mitochondria are evident [10] , [11] , [12] , [13] . Finally, analyses in Drosophila indicated that the expression of genes that localize to the mitochondria is responsive to engineered deletions that decreased rDNA CN [8] . Hence, these observations raise the expectation that the cross-talk between the rDNA dosage and mitochondrial abundance might be manifested across genotypes in natural populations. 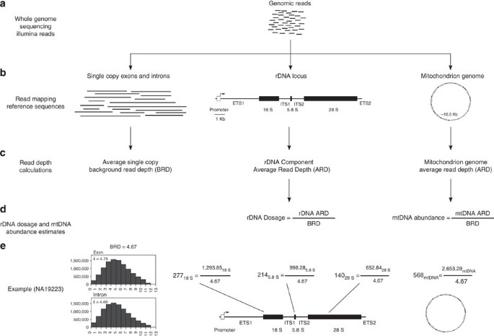Figure 1: Experimental procedure to estimate rDNA dosage and mtDNA abundance from short-read whole-genome sequence data. (a,b) Genomic reads were quality trimmed and mapped against a panel of single-copy exons and introns, the rDNA locus and the mitochondrion genome. (c) BRD, representing the average read depth of a single-copy DNA sequence, was calculated from the exon and intron reference set. Average read depth (ARD) of the rDNA locus and mitochondrion genome was calculated. (d) rDNA and mtDNA ARD values were normalized by BRD to estimate dosage and abundance, respectively. (e) An example of rDNA dosage and mtDNA estimations for sample NA19223 and correlation of BRD estimates using our sets of single-copy exon and intron across samples. Figure 1: Experimental procedure to estimate rDNA dosage and mtDNA abundance from short-read whole-genome sequence data. ( a , b ) Genomic reads were quality trimmed and mapped against a panel of single-copy exons and introns, the rDNA locus and the mitochondrion genome. ( c ) BRD, representing the average read depth of a single-copy DNA sequence, was calculated from the exon and intron reference set. Average read depth (ARD) of the rDNA locus and mitochondrion genome was calculated. ( d ) rDNA and mtDNA ARD values were normalized by BRD to estimate dosage and abundance, respectively. ( e ) An example of rDNA dosage and mtDNA estimations for sample NA19223 and correlation of BRD estimates using our sets of single-copy exon and intron across samples. Full size image Here we develop a method for assessing rDNA dosage and mitochondria abundance using local variation in coverage depth in short-read whole-genome DNA sequence data ( Fig. 1 ). We apply this methodology to human whole-genome sequencing data [14] and investigate the extent of variation in rDNA dosage (the number of rDNA copies present in a given genome) and mitochondria DNA abundance (the number of mitochondrial genomes present in a cell). Estimates of rDNA dosage and mitochondria (mitochondrial DNA (mtDNA)) abundance are combined with gene expression (GE) estimates from RNA-seq data to reveal the functional consequences of rDNA dosage variation. Our analysis sheds new light on the diverse functional roles of the rDNA loci and uncovers coordinated variation between the rDNA loci and global GE, as well as mitochondrial abundance. The associations are manifested in the context of naturally occurring variation among individuals. Estimation of rDNA dosage Local variation in read depth has been benchmarked as a reliable method for the identification and quantification of CNV [15] , [16] . We modified the approach to quantify dosage of the rRNA encoding loci, as the read depth coverage of the rDNA components relative to baseline read depth of single copy sequences (see Fig. 1 for methodological pipeline). Reads for each sample were quality trimmed and mapped against the reference (i) panel of single copy exons (12,453 exon totaling 13.09 Mb), (ii) panel of single copy introns (1,131 introns totaling ~1.27 Mb), (iii) 45S rDNA locus (the locus containing the 18S, 5.8S and 28S rRNA encoding genes) [17] and (iv) mitochondrion genome ( Fig. 1 , see Methods). Per-base read depth values were normally distributed and sample-specific sequence read depth was estimated by the mean base coverage ( Fig. 1e ). The average per-base single copy exon and single copy intron was used as a proxy for the background read depth (BRD). We focus subsequent analyses on 168 individuals from 2 populations with genomic coverage >4 × ( Supplementary Table 1 ). Our calculation of BRD produced nearly identical estimates of genomic coverage for both exon and intron reference data sets ( r 2 =0.99, P =1.5 × 10 −173 ; Supplementary Fig. 1 ). BRD ranged from 4.7 to 16.2 × and, importantly, was not correlated with dosage of any rDNA component. Average per-base read depth of rDNA sequences was normalized by the BRD to estimate rDNA dosage ( Fig. 1 , see Methods). Several analyses validate our rDNA dosage estimates. First, we measured CN for six unrelated genes that were previously characterized [16] (see Methods). Our results strongly agree with previous estimates across all six genes (average r 2 =0.88; Supplementary Fig. 2 ), including the two genes with experimental validation ( CCL3L1 : r 2 =0.91, P =2.3 × 10 −43 and TBC1D3F : r 2 =0.81, P =9.8 × 10 −30 ; Supplementary Fig. 2a,b ). Second, we investigated whether sequence similarity between rDNA components might confound estimates. We observed complete lack of sequence similarity between rDNA components using either BLAST or ClustalW alignments. Conversely, each rDNA component is highly conserved between humans and mouse (Pairwise nucleotide identity: 18S=100%, 5.8S=99% and 28S=86%). Indeed, inspection of reads mapping to the rDNA revealed that no reads mapped to multiple rDNA components (see Methods; Supplementary Fig. 3 ). These analyses indicate that the rDNA components did not interfere with one another during read mapping and point to robust computational estimates of rDNA dosage. Third, estimates of rDNA dosage could be confounded if reads that map to the rDNA loci also map to pseudogenes at alternative regions of the genome. To address the issue, we extracted reads that mapped to each component of the reference rDNA locus and mapped those ‘rDNA reads’ against the reference GRCh37 (hg19) human genome (see Methods; Fig. 2 ). The reference genome includes chromosomes and all supercontigs that have not been assigned a chromosomal location. The chromosomal regions containing nucleolar organizing regions are masked in the reference genome. The procedure was independently performed for each of the 168 samples. As expected, the vast majority of 45S rDNA reads mapped to a single supercontig that harbours the 45S rDNA locus (GL000220.1; 18S: 87.41%, 5.8S: 98.3% and 28S: 94.4%; Fig. 3a ). Hence, for each individual, we used the percentage of reads mapping to the expected chromosomes and contigs as a correction factor to obtain the best estimates of 18S, 5.8S and 28S dosage. The correction had minor but beneficial effect on individual estimates and resulted in a slightly higher correlation for 18S versus 5.8S ( r =0.80 versus r =0.79), and identical correlations for 28S versus 18S and 28S versus 5.8S. Interestingly, the majority of the ~13% of 18S reads, which did not map to GL000220.1 supercontig, mapped to a small (~600 bp) region of chromosome 21 (9,826,921–9,827,532; Fig. 3b ). BLAST results indicate that this region, and its flanking regions, share homology with ETS1 and 18S but with no other rDNA elements ( Fig. 3b ). This suggests that the region is probably a truncated and pseudogenized rDNA array. 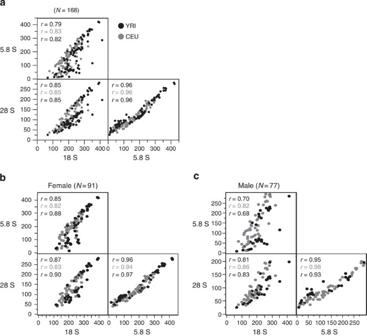Figure 2: Dosage estimates for the three components of the 45S rDNA are highly correlated with one another. (a) Pairwise Pearson’s correlation (r) for the 45S rDNA components (N=168). For all correlationsP-value ≤2 × 10−37. Grey and black points represent the CEU and YRI populations, respectively. (b,c) Correlations are consistent when stratified by sex. For all comparisons, the bold Pearson value corresponds to the combined data set, while the grey and black Pearson values represent the CEU and YRI populations, respectively. Dosage is estimated as the number of rDNA copies per diploid genome. Figure 2: Dosage estimates for the three components of the 45S rDNA are highly correlated with one another. ( a ) Pairwise Pearson’s correlation ( r ) for the 45S rDNA components ( N =168). For all correlations P -value ≤2 × 10 −37 . Grey and black points represent the CEU and YRI populations, respectively. ( b , c ) Correlations are consistent when stratified by sex. For all comparisons, the bold Pearson value corresponds to the combined data set, while the grey and black Pearson values represent the CEU and YRI populations, respectively. Dosage is estimated as the number of rDNA copies per diploid genome. 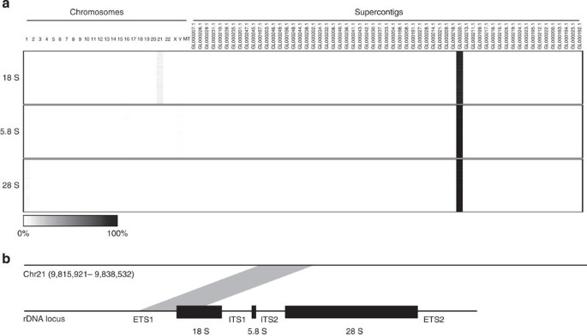Figure 3: rDNA reads map to the expected supercontigs and reveal a truncated rDNA array on chromosome 21. (a) Heat map depicting the percentage of reads mapping to each chromosome and supercontig of the human genome (hg19). For each individual (N=168), the colour of the heat map corresponds to the percentage of rDNA reads mapped to each chromosome or supercontig, where white is zero and black is 100%. Theyaxis represents each individual and thexaxis represents chromosomes and supercontigs. The vast majority of rDNA reads map to the rDNA locus containing supercontig (GL000220.1). The fraction of reads correctly mapped to the expected supercontig was used as a correction factor. (b) Region of chromosome 21 (9,815,921–9,838,532) to which 18S reads map. The grey shaded area represents the region of homology between the segment of chromosome 21 and the rDNA locus. Full size image Figure 3: rDNA reads map to the expected supercontigs and reveal a truncated rDNA array on chromosome 21. ( a ) Heat map depicting the percentage of reads mapping to each chromosome and supercontig of the human genome (hg19). For each individual ( N =168), the colour of the heat map corresponds to the percentage of rDNA reads mapped to each chromosome or supercontig, where white is zero and black is 100%. The y axis represents each individual and the x axis represents chromosomes and supercontigs. The vast majority of rDNA reads map to the rDNA locus containing supercontig (GL000220.1). The fraction of reads correctly mapped to the expected supercontig was used as a correction factor. ( b ) Region of chromosome 21 (9,815,921–9,838,532) to which 18S reads map. The grey shaded area represents the region of homology between the segment of chromosome 21 and the rDNA locus. Full size image rDNA dosage is highly polymorphic Diploid rDNA dosage was quantified for each coding component of the rDNA locus (18S, 5.8S and 28S regions). Diploid rDNA dosage for each component ranged from 67 to 412 for 18S ( copies), 9 to 421 for 5.8S ( copies) and 26 to 282 for 28S ( copies). Further, the components of the 45S rDNA locus were significantly and strongly correlated with one another ( Fig. 2 ; N =168; 18S versus 5.8S: Pearson’s r =0.79, P =2 × 10 −37 , 18S versus 28S: r =0.85, P =2 × 10 −47 and 5.8S versus 28S: r =0.96, P =1 × 10 −95 ). These patterns were consistent between populations and between sexes ( Fig. 2 ). The associations are expected due to the close physical linkage between the components of the 45S rDNA array. Nevertheless, abnormally rearranged rDNA loci might contribute to variability in dosage between rDNA components [18] , [19] , [20] and might account for the weaker association between the 18S and the 35S components (5.8S and 28S). In terms of the range of our computational rDNA dosage measurements, our results are consistent with previous experimental estimates of 45S dosage measured by the cumulative physical size of the rDNA clusters [21] , [22] . Collectively, the data point to substantial variation across individuals. Loci with dosage variation might display variable levels of population differentiation ranging from an absence of population differentiation to high levels of differentiation [16] . To address the issue for the rDNA loci, we estimated V ST values between Ceph (CEU) and Yoruban (YRI) populations. We observe no evidence for population differentiation within the rDNA loci (18S V ST =0.09, 5.8S V ST <0.001 and 28S V ST =0.01; Fig. 4a–c ). Principal component analyses (PCAs) of the rDNA dosage components further reinforce the conclusion that these populations are not differentiated in regards to rDNA dosage ( Fig. 4d,e ). 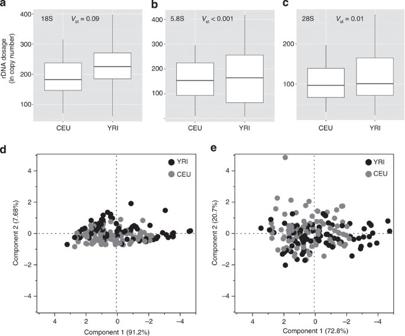Figure 4: rDNA dosage do not display population differentiation. VSTvalues for the (a) 18S, (b) 5.8S and (c) 28S rDNA components (N=168). CN is depicted on theyaxis, while the CEU and YRI populations are shown on thexaxis. Box plots display the median, the 25th and 75th percentiles, and maximum and minimum. PCA analysis of (d) 45S rDNA component (18S, 5.8S and 28S) CNs, (e) 45S and mtDNA abundance (N=168). Thexandyaxes represent the first two principal components. Grey and black symbols represent the CEU and YRI individuals, respectively. Figure 4: rDNA dosage do not display population differentiation. V ST values for the ( a ) 18S, ( b ) 5.8S and ( c ) 28S rDNA components ( N =168). CN is depicted on the y axis, while the CEU and YRI populations are shown on the x axis. Box plots display the median, the 25th and 75th percentiles, and maximum and minimum. PCA analysis of ( d ) 45S rDNA component (18S, 5.8S and 28S) CNs, ( e ) 45S and mtDNA abundance ( N =168). The x and y axes represent the first two principal components. Grey and black symbols represent the CEU and YRI individuals, respectively. Full size image The rDNA is a trans -regulatory eQTL Recent data suggested that rDNA deletions might disrupt GE levels and chromatin states in Drosophila [8] , [23] . Substantial association in dosage among unlinked loci further lends support to the hypothesis that variability at the rDNA loci might have functional relevance for GE states across the genome. Accordingly, we hypothesized that rDNA dosage might function as expression quantitative trait loci (eQTL) modulating natural variation in GE levels among individuals. To address the issue, we cross-referenced our estimates of rDNA dosage with genome-wide GE data from the HapMap project [24] , [25] (see Methods). The combined data set consists of 97 individuals with corresponding rDNA dosage estimates and whole-genome expression data from lymphoblastoid cell lines ( Supplementary Table 1 ). Genome-wide association between rDNA dosage estimates and GE levels was calculated for each rDNA component independently using Pearson’s correlation and, formally, through mixed linear models ( Fig. 5 ). These analyses revealed highly statistically significant and comparable associations across the 18S, 5.8S and 28S rDNA components (as expected due to strong rDNA dosage correlations between components; Fig. 5a ). To obtain a single best estimate for the 45S rDNA we combined estimates using Fisher’s combined probability method (see Methods). The procedure identified 1,371 genes whose expression was significantly associated with rDNA dosage ( P <0.01; false discovery rate (FDR)=0.06; Fig. 3b ), 198 of which remain highly significant after a stringent Bonferroni correction ( P <6.4 × 10 −6 ; FDR=0.0002; Fig. 3b ). No chromosomal bias of significantly correlated genes was observed when tested against the distribution due to chance ( χ 2 goodness-of-fit, degree of freedom (DF)=22, P more-stringent =0.48 and P less-stringent =0.77). Surprisingly, positive associations are significantly more abundant than negative associations and make up >70% of correlated genes ( χ 2 goodness-of-fit, DF=1, P more-stringent =4.3 × 10 −18 and P less-stringent =9.8 × 10 −5 ). It is worth noting that we performed several analyses to ascertain the robustness of our inferences to confounders due to population structure, uncertainty in mRNA estimates and hidden sources of expression variation (see Methods). Most conservatively, we also identified rDNA-responsive genes independently within the CEU and YRI populations ( Fig. 5c–e ), and investigated patterns in an independently collected GE data set for the CEU population (see below). These analyses are in good agreement with one another (see section below), reinforce previous observations in Drosophila [8] and indicate that rDNA dosage is a major determinant of naturally occurring genome-wide GE variation in humans. 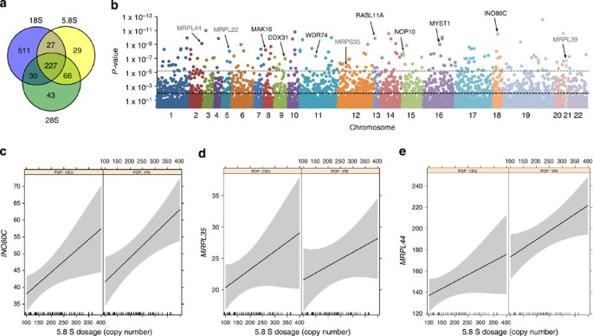Figure 5:rDNA dosage is a majortrans-regulatory eQTL (Ribo-eQTL). (a) Independent associations between components of the 45S rDNA share significant overlap. Venn diagram of genes significantly correlated (P-value <0.01) with rDNA dosage and GE. (b) Manhattan plot of genome-wide association results between 45S rDNA CN and GE. Colours represent chromosomes and the Fisher’s combined Pearson’s correlation probability for the 18S, 5.8S and 28S rDNA components is depicted on theyaxis. The dotted black line represents theP-value significance thresholds of 0.01, while the grey line represents the Bonferroni multiple test correctedP-value significance threshold of 6.4 × 10−6. Examples of specific genes are labelled. (c–e) Examples of associations between 5.8S dosage and GE in CEU and YRI populations. (c)INO80Cis a chromatin modifying gene, while (d) MRPL35 and (e) MRPL44 are mitochondrial ribosomal genes. rDNA dosage and GE levels are represented on thexandyaxes, respectively. The grey area represents the 95% intervals for the linear coefficients. Figure 5: rDNA dosage is a major trans -regulatory eQTL (Ribo-eQTL). ( a ) Independent associations between components of the 45S rDNA share significant overlap. Venn diagram of genes significantly correlated ( P -value <0.01) with rDNA dosage and GE. ( b ) Manhattan plot of genome-wide association results between 45S rDNA CN and GE. Colours represent chromosomes and the Fisher’s combined Pearson’s correlation probability for the 18S, 5.8S and 28S rDNA components is depicted on the y axis. The dotted black line represents the P -value significance thresholds of 0.01, while the grey line represents the Bonferroni multiple test corrected P -value significance threshold of 6.4 × 10 −6 . Examples of specific genes are labelled. ( c – e ) Examples of associations between 5.8S dosage and GE in CEU and YRI populations. ( c ) INO80C is a chromatin modifying gene, while ( d ) MRPL35 and ( e ) MRPL44 are mitochondrial ribosomal genes. rDNA dosage and GE levels are represented on the x and y axes, respectively. The grey area represents the 95% intervals for the linear coefficients. Full size image Expression responses to rDNA dosage are functionally coherent Ribosome biogenesis involves a complex and concerted effort from ~80 ribosomal proteins and the hundreds of other ribosomal associated proteins, including transcription factors, enzymes, chaperones and nuclear export complexes [26] . The ribosome is assembled in the nucleolus, a dense nuclear compartment first recognized over two centuries ago [27] , [28] , and rDNA dosage might be particularly relevant for regulating genes functionally associated with this nuclear organelle. In agreement with our expectations, several genes whose expression is significantly and positively correlated with rDNA dosage are associated with the nucleolus. These include the following: RASL11A and DDX31 , which are known regulators of rRNA expression; MAK16 , which is involved in 60S ribosome biogenesis; NOP2 , which is a putative methyltransferase, regulates the 25S rRNA and influences 60S assembly in yeast; NOP10 , which is a small nucleolar ribonucleoprotein that may facilitate small nucleolar ribonucleoprotein assembly; and WDR74 , which plays a crucial role in the processing and maturation of 18S rRNA [29] , [30] ( Fig. 5b ). To further identify functionally coherent classes, we used the Gene Ontology (GO) annotation to categorize genes that are sensitive to rDNA dosage (see Methods). In agreement with our expectations, we observed that genes whose expression is positively associated with rDNA dosage are coherently clustered across several GO categories that are functionally related to the rDNA ( Supplementary Table 2 ). Specifically, we observed significant enrichments in candidates localized to the nucleolus ( P =9.8 × 10 −4 ), ribonucleoprotein complex ( P =2.2 × 10 −6 ), ribosome ( P =2.4 × 10 −4 ), mitochondrial ribosome ( P =3.0 × 10 −4 ) and spliceosomal complex ( P =6.4 × 10 −4 ; Fig. 6 and Supplementary Table 2 ). The analyses also highlight significant enrichments in the processes of spliceosomal sn RNP assembly ( P =8.5 × 10 −4 ), RNA metabolism ( P =9.3 × 10 −4 ), nc RNA metabolism ( P =9.6 × 10 −4 ) and response to virus ( P =6.9 × 10 −4 ; Fig. 6a and Supplementary Table 2 ). Furthermore, the analyses point to a distinct set of genes negatively associated with rDNA dosage, with significant enrichment in candidates localized to the endoplasmatic reticulum ( P =1.8 × 10 −5 ; Fig. 6a ). Finally, consistent with the suggestion that rDNA dosage may alter genome-wide chromatin states [8] , several genes with epigenetic roles in chromatin modification showed significant association with rDNA dosage, including CBX1 (HP1 β), CTCF , CDYL2 , MYST1 , RASL11A , CENPA , KTI12 , INO80C and KDM4B ( Fig. 5b,c ). Notably, HP1 β is known to associate with the nucleolus and play a role in the transcription of ribosomal proteins [31] and CTCF also localizes in the nucleolus and influences the chromatin state of rDNA arrays [32] . Altogether, the data highlight coherent genomic responses to rDNA dosage, including a greater expression of ribosomal-associated proteins in response to higher rDNA dosage. 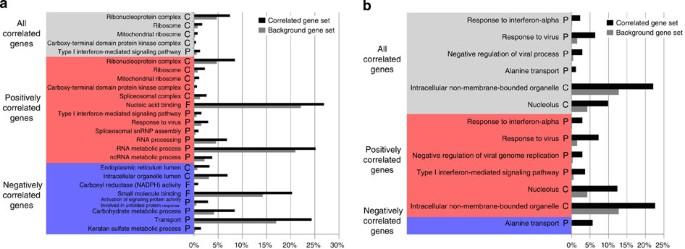Figure 6: rDNA dosage is associated with the expression of functionally coherent genes. GO functional enrichment analysis of correlated genes for significance thresholds of (a)P<0.01 and (b)P<6.4 × 10−6(N=97). Redundant GO terms were reduced for clarity of display (seeSupplementary Table 1for complete GO term enrichment). Grey, red and blue shaded boxes represent GO term enrichment for all correlated, positively correlated and negatively correlated genes, respectively. Black and grey bars represent the percentages of correlated and background genes classified in each GO term, respectively. For all enriched GO termsP-value <1 × 10−3. Figure 6: rDNA dosage is associated with the expression of functionally coherent genes. GO functional enrichment analysis of correlated genes for significance thresholds of ( a ) P <0.01 and ( b ) P <6.4 × 10 −6 ( N =97). Redundant GO terms were reduced for clarity of display (see Supplementary Table 1 for complete GO term enrichment). Grey, red and blue shaded boxes represent GO term enrichment for all correlated, positively correlated and negatively correlated genes, respectively. Black and grey bars represent the percentages of correlated and background genes classified in each GO term, respectively. For all enriched GO terms P -value <1 × 10 −3 . Full size image Additional analyses validate the functional coherence of loci that are sensitive to rDNA dosage. First, we observed that independent estimates are in good agreement between CEU and YRI populations, with the associations (genome-wide correlation coefficients) significantly correlated between populations (5.8S: r =0.14, P =7 × 10 −34 and 28S: r =0.19, P =5 × 10 −36 ). Indeed, genes similarly associated with the 5.8S in both CEU and YRI were enriched in targets that localize to the nucleolus ( P =1.93 × 10 −4 ), the ribosome ( P =4.36 × 10 −4 ) and that belonging to the endoplasmatic reticulum membrane protein complexes ( P =7.87 × 10 −4 ). Using this approach we identified, for instance, RASL11A , INO80C and MRPL44 as responsive to rDNA dosage (highlighted in Fig. 5b,c,e ). These observations indicate that the major functional associations can be replicated independently within each population. Second, we performed association analysis on a subset of 27 overlapping CEU individuals for which RNA-seq data were generated from another study and processed through the same analysis pipeline [33] , [34] . We observed good agreement between expression values for biological replicates used between the studies (average Pearson correlation ( r ) between expression values=0.87). Despite the much smaller size of the Cheung et al . [33] data set, the association between rDNA dosage and GE were significantly correlated between studies (correlations between the strength of the association uncovered with expressed data from the Cheung et al . [33] study and from the Montgomery e t al. [24] study: 18S: r =0.13, P =5 × 10 −28 ; 5.8S: r =0.23, P =6 × 10 −73 ; 28S: r =0.21, P =1 × 10 −58 ; mtDNA: r =0.47, P =4 × 10 −301 ) and functional analysis similarly suggested an enrichment in candidates that localize to the mitochondria (mitochondrial part and mitochondrion; P <8. × 10 −4 for both categories). Lastly, patterns of functional enrichment were highly concordant between the PCA normalized and non-PCA normalized CEU expression data ( Supplementary Tables 3 and 4 ). Altogether, our results with independently measured expressions levels from the same cells and with replication across populations lend support to the conclusion that the trans -regulatory consequence of rDNA dosage is pervasive and coherently manifested. rDNA dosage is negatively associated with mtDNA abundance Several studies indicate a close relationship between the rDNA arrays, ribosomal biogenesis and the mitochondria [10] , [11] , [12] , [13] . For instance, recent evidence points to the import of 5S rRNAs into the mitochondria through a highly regulated process [35] , [36] . Moreover, tight regulation of nuclear transcription ensures proper mitochondrial biogenesis [11] , [13] . As such, functional cross-talk between the rDNA dosage and the mitochondria might be manifested in natural populations. Indeed, the association between rDNA gene dosage and mitochondria is consistent with the overrepresentation of mitochondrial ribosome ( Fig. 6a ) genes in the set of candidates positively associated with rDNA dosage. Furthermore, the expression of 25 of the 50 nuclear genes encoding mitochondrial proteins analysed was significantly positively associated with rDNA dosage (at the P -value threshold of 0.01; see ‘ MRP ’ genes in Fig. 5 ). Altogether, the data indicate that rDNA gene dosage might influence mitochondrial-related processes. To address this issue, we quantified mtDNA abundance using an approach similar to that used for estimating rDNA dosage ( Fig. 1 , see Methods). Accordingly, we observed ~4-fold variation in mtDNA abundance among individuals, ranging from 226 to 1,074 mtDNA per diploid nuclear genome. Remarkably, mtDNA abundance was significantly negatively associated with dosage of all rDNA components ( n =168; mtDNA versus 18S: Pearson’s r =−0.29, P =1.3 × 10 −4 , mtDNA versus 5.8S: Pearson’s r =−0.34, P =5.4 × 10 −6 and mtDNA versus 28S: r =−0.36, P =1.2 × 10 −6 ; Fig. 7a ). Our results point towards interactions between rDNA and the mitochondria that is manifested across human genotypes. We find that rDNA dosage (i) influences the expression of mitochondrial-related genes ( Figs 5b,d,e and 6a ) and (ii) is negatively associated with mtDNA abundance ( Fig. 7a ). These results might reflect the synchronization of GE between the nuclear and mitochondrial genomes in a concerted effort to control proper levels of protein production for mitochondria assembly and intracellular homeostasis. Retrograde signalling is an essential mechanism in which organelles communicate with the nucleus to convey a response from fluctuating environmental or cellular conditions [10] . Indeed, we found that genes whose expression is negatively correlated with rDNA dosage were functionally enriched for carbonyl reductase (NADPH) activity ( Fig. 6a ). This observation is particularly noteworthy because NADPH oxidases are involved in the mitochondria–nucleus cross-talk [10] . 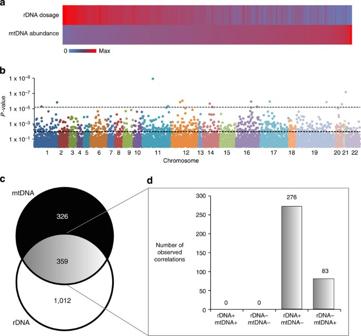Figure 7: rDNA dosage and mitochondrial DNA abundance are inversely correlated. (a) rDNA CN and mtDNA abundance are inversely correlated. rDNA dosage (average CN of the 18S, 5.8S and 28S components) and mtDNA abundance are depicted for each of the 168 individuals. Blue and red correspond to zero and the measurement maximum, respectively. Individuals are sorted in ascending order of mtDNA abundance (N=168). (b) Manhattan plot of genome-wide association between mtDNA CN and GE (N=97). The dotted black line represents the significance threshold ofP<0.01, while the grey line represents the Bonferroni multiple test correctedP-value significance threshold of 6.4 × 10−6. (c) Venn diagram showing significant overlap (grey) between genes whose expression is correlated with mtDNA (black) or rDNA (white). (d) All genes displaying association with both mtDNA and rDNA are inversely correlated. Thexaxis represents the class of each overlapping correlated gene; ‘+’ and ‘−’symbols depict positively and negatively correlated genes, respectively, and theyaxis provides the frequency of each occurrence. Figure 7: rDNA dosage and mitochondrial DNA abundance are inversely correlated. ( a ) rDNA CN and mtDNA abundance are inversely correlated. rDNA dosage (average CN of the 18S, 5.8S and 28S components) and mtDNA abundance are depicted for each of the 168 individuals. Blue and red correspond to zero and the measurement maximum, respectively. Individuals are sorted in ascending order of mtDNA abundance ( N =168). ( b ) Manhattan plot of genome-wide association between mtDNA CN and GE ( N =97). The dotted black line represents the significance threshold of P <0.01, while the grey line represents the Bonferroni multiple test corrected P -value significance threshold of 6.4 × 10 −6 . ( c ) Venn diagram showing significant overlap (grey) between genes whose expression is correlated with mtDNA (black) or rDNA (white). ( d ) All genes displaying association with both mtDNA and rDNA are inversely correlated. The x axis represents the class of each overlapping correlated gene; ‘+’ and ‘−’symbols depict positively and negatively correlated genes, respectively, and the y axis provides the frequency of each occurrence. Full size image Mitochondrial DNA abundance and genome-wide expression Finally, we evaluated the relationship between mtDNA abundance and nuclear GE, and identified 685 genes significantly correlated with mtDNA abundance ( P <0.01, FDR=0.07), 14 of which remained significant after a stringent Bonferroni-corrected threshold ( Fig. 7b ). Interestingly, over half the genes whose expression is associated with mtDNA abundance (359 genes) also showed significant association with rDNA dosage ( P <0.01; Fig. 7c ). The overlap was substantially greater than expected by chance ( χ 2 goodness-of-fit, DF=1, P =3.9 × 10 −107 ). However, in contrast to that observed with rDNA dosage, negative associations between mtDNA abundance and nuclear GE were significantly more prevalent than positive associations ( χ 2 goodness-of-fit, DF=1, P =1.8 × 10 −6 ). Indeed, all of the overlapping genes were inversely associated (that is, positively correlated with rDNA dosage and negatively correlated with mtDNA abundance, or negatively correlated with rDNA dosage and positively correlated with mtDNA abundance; Fig. 7d ). All eight of the mitochondrial ribosomal protein-encoding genes in the overlapping data set were positively correlated with rDNA dosage and negatively correlated with mtDNA abundance. None of the nuclear ribosomal protein-encoding genes was correlated with both the rDNA dosage and mtDNA abundance. Hence, the data indicate a balanced relationship between rDNA dosage and mtDNA abundance that is manifested as an inverse association between these two elements in natural populations and divergent associations with genome-wide levels of expression. Interestingly, we also observed significant correlations between both rDNA dosage (positive) and mtDNA abundance (negative) with the mitochondrial transcription termination factor 3 ( MTERF ). This protein regulates mitochondrial transcription and mitochondrial ribosome biogenesis [12] . These results suggest tight regulatory relationship between rDNA dosage, GE of ribosomal proteins and mtDNA abundance, which emerge in the context of naturally occurring variability among individuals ( Fig. 8 ). 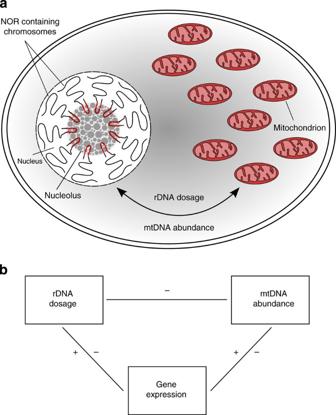Figure 8: Model summary with interactions between rDNA dosage and mtDNA abundance. (a) Within the eukaryotic nucleus, variable sized nucleolar organizing regions (NORs) localize to the nucleolus, associate with the expression of hundreds of genes and negatively correlate with mtDNA abundance. (b) Qualitative summary of the sign (negative or positive) of the associations herein uncovered. rDNA dosage and mtDNA abundance display inverse associations with GE (that is, genes with expression positively correlated with rDNA dosage and negatively correlated with mtDNA abundance or gene with expression negatively correlated with rDNA dosage and positively correlated with mtDNA abundance). These associations emerge at the population level as naturally occurring variation among individuals. Figure 8: Model summary with interactions between rDNA dosage and mtDNA abundance. ( a ) Within the eukaryotic nucleus, variable sized nucleolar organizing regions (NORs) localize to the nucleolus, associate with the expression of hundreds of genes and negatively correlate with mtDNA abundance. ( b ) Qualitative summary of the sign (negative or positive) of the associations herein uncovered. rDNA dosage and mtDNA abundance display inverse associations with GE (that is, genes with expression positively correlated with rDNA dosage and negatively correlated with mtDNA abundance or gene with expression negatively correlated with rDNA dosage and positively correlated with mtDNA abundance). These associations emerge at the population level as naturally occurring variation among individuals. Full size image All aspects of cellular growth and development are dependent on ribosome biogenesis and protein synthesis. rRNA molecules make up the majority of eukaryotic ribosomes and, unlike mRNA transcripts, cannot be recycled through multiple rounds of amplification via translation. Hence, high CN rDNA arrays are expected to provide a sufficient source of cellular rRNAs to maintain a viable pool of rRNA molecules [37] . It is not surprising that sequence and structural rDNA polymorphisms can have drastic phenotypic consequences and association with disease [7] , [38] . Here we provide computational estimates of rDNA dosage and mtDNA abundance across hundreds of human genomes. Our analyses show abundant variation in rDNA dosage with regulatory properties (Ribo-eQTL) that functionally interact with genome-wide GE and mtDNA abundance. In spite of the high level of sequence and functional conservation of rRNA molecules among eukaryotes, CN of the rDNA locus is variable both within and between species [38] . Indeed, eukaryotic genomes display dramatic differences in rDNA dosage ranging from as few as ~20 to as many as 20,000 copies [39] . Extensive epigenetic regulation of the rDNA loci further contributes to the complexity, with greater rDNA dosage not directly equating to higher expression levels of rRNA transcripts. Accordingly, an estimated ~50% of rDNA loci are transcriptionally inactivated [40] and further, total rRNA transcription can be compensated by upregulating individual rDNA loci rather than the activation of additional copies of the locus [41] . One established notion is that the functionally redundant rDNA copies in the genome provide more resources to transcribe rRNAs than what is typically required for ribosome biogenesis in actively growing cells [38] . However, lower limits of rDNA dosage are evident. For example, in chicken strains, fewer than half of wild-type rDNA dosage caused embryonic lethality [42] , while in yeast, isolates with experimentally reduced rDNA dosage experience a gradual return to original levels over time [43] . On the other hand, upper limits placing boundaries of rDNA dosage might be less sharply defined. Rapid amplification of the locus has long been well documented in somatic tissues of fruitflies that inherit reduced rDNA arrays [44] , [45] , [46] , [47] , and an upwards of 10,000-fold amplification of the rDNA has been well described in amphibians oocytes [48] , [49] . These observations, along with others, indicate that somatic gene amplification and selection might contribute to shaping rDNA dosage [38] and that molecular models for the trans -regulatory effects of rDNA dosage need to be refined. In any circumstance, the associations between GE and dosage variation in the rDNA might point to molecular requirements and trade-offs that place boundaries on the range of rDNA dosage typically observed. We expect that, via the alteration of epigenetic states across the genome, these trade-offs might contribute to intragenomic adaptations with relevance to shaping optimal ranges for rDNA dosage. Our results also show that polymorphic dosage variation in the rDNA locus interacts with the remaining of the genome beyond the production of rRNAs for ribosome biogenesis. Epigenetic models of chromatin dynamics [50] that postulate a finite supply of dosage-sensitive chromatin regulators and DNA-binding proteins in the nucleus might explain the trans -regulatory modulation by Ribo-eQTL. These could involve, for instance, differential recruitment of chromatin-modifying proteins to rDNA arrays with variable CN. Disproportional binding to rDNA locus might result in altered concentrations throughout the rest of the genome, thereby effecting genome-wide chromatin environments and transcription rates [8] , [51] , [52] , [53] . The observation that rDNA dosage is correlated with the expression of several proteins that modify the chromatin ( Fig. 5b,c ) is consistent with such a model. If these proteins are sequestered through preferentially binding to elements of the rDNA loci [42] , [43] , limited availability elsewhere in the genome might be expected to cause upregulation of GE in individuals with greater rDNA dosage. Such source-sink mechanisms might explain the strong biases for positive associations between GE and rDNA dosage. Our study revealed substantial variation in rDNA dosage among individuals, ranging from as low as approximately ten to hundreds of copies that function as a major trans -regulatory modifier (Ribo-eQTL) of genome-wide expression and mitochondria abundance ( Fig. 8 ). Limited availability of transcription factors or chromatin regulators required for rRNA transcription and for maintaining the epigenetic architecture of the rDNA loci might be one mechanism to account for genome-wide consequences of rDNA dosage. Our findings uncover a novel source of functional genomic variation in rDNA dosage that is hypervariable and revealed through the expression of functionally coherent sets of gene across the entire genome. They raise the question of how pervasive these consequences might be to other traits, including organismal fitness, cellular adaptation and disease phenotypes. Several examples of adaptive CNV are present in human populations [54] . In line with these patterns, variation in rDNA dosage might conceivably provide a molecular mechanism for cellular homeostasis, as well as a rapid and reversible source of variation for adaptation at the cellular and organismal levels. Human population genome data Raw fastq whole-genome DNA Illumina sequence reads for individuals with estimated coverage >5 × were obtained from the 1,000 Genomes Project FTP site ( http://1000genomes.org ) [14] . Approximate sequence read coverage was estimated pre-mapping by multiplying read length by read count. We focused on individuals from the CEU and YRI populations, as they represented populations with substantial, high-coverage samples. We quality trimmed reads from each sample using Trim Galore ( http://www.bioinformatics.babraham.ac.uk/projects/trim_galore/ ). Residual adapter sequences were removed from reads, and reads were trimmed such that they contained a minimum quality score of 20 at each nucleotide position. Trimmed reads shorter than 50 nucleotides were discarded. Reference sequences The consensus 43 Kb human rDNA reference sequence was obtained from GenBank (accession: U13369 ) [17] . We modified this sequence to include a ~17.65-kb region of the rDNA locus extending 2 kb upstream of the core promoter region to 2 kb downstream of the ETS2 region ( Fig. 1b ). The entire human mitochondrion genome was downloaded from the NCBI Reference Sequence Database (accession: NC_012920.1) [55] . The complete human exon reference was downloaded from The European Bioinformatics Institute ( ftp://ftp.ebi.ac.uk/pub/databases/astd/current_release/human/9606_exons.fa.gz ). To retain putative single-copy exons, we performed several layers of filtering. First, exons with significant BLAST hits ( E -value <1 × 10 −6 ) [56] to any other exons were removed to reduce potentially ambiguous regions. Second, only the largest exon of each gene was retained to avoid mapping to alternatively transcribed exons with overlapping regions. Third, only exons ⩾ 300 bp were retained to reduce mapping biases to short target regions. Our final single-copy exon reference data set consisted of 12,453 sequences. The complete set of human introns was downloaded from the UCSC Genome Table Browser. We performed similar, but additional, filtering as the exons to obtain a reliable set of single copy introns: (i) introns with significant BLAST hits ( E -value <1 × 10 −6 ) to any other introns were removed, (ii) only the largest intron of each gene was retained, (iii) only the first intron located within 10 kb of any other intron was retained, (iv) only introns ⩾ 300 bp were retained, (iv) only introns ≤10 kb were retained. This filtering resulted in an intron data set consisting of 1,131 introns. Read mapping Filtered read sets for each sample were mapped against the reference rDNA locus, mitochondrion genome and sets of single-copy exons and introns using Bowtie2 v2.0.5 (ref. 57 ). Reads were mapped in unpaired fashion using the ‘sensitive’ preset (full command line parameters: --end-to-end -D 15 -R 2 -L 22 -i S,1,1.15). Mapping output was converted to sorted bam format using the samtools (v0.1.18) ‘view’ and ‘sort’ functions, respectively [58] . Background read depth estimation BRD was calculated for each sample and was used as a normalizing factor to estimate rDNA component dosage and mtDNA abundance ( Fig. 1c–e ). Per-base BRD was independently calculated from the exon and intron sorted bam mapping output files using the samtools ‘depth’ function [58] . To correct for artificial mapping reduction in the beginning and end of reference sequences, per-base depth values from the first and last 108 bp (longest read length in data set) were excluded. For each sample, we excluded read depth values in the upper 5% of the distribution. Exon and intron BRD estimates were nearly identical ( r 2 =0.99; Supplementary Fig. 1 ). Hence, we used the average of the two values to represent consensus BRD. rDNA dosage and mtDNA abundance estimation Consensus BRD was used as a normalizing factor to represent the read depth of an autosomal locus with a diploid CN of two. Average read depth of each rDNA component was also calculated using the samtools ‘depth’ function ( Fig. 1c ). For each sample, rDNA component dosage was calculated as: where ARD is the average read depth across all sites in the rDNA component and BRD is the background read depth. Stability in CN variable loci has been demonstrated in DNA extracted from lymphoblastoid cell lines versus whole blood [59] , [60] , [61] . We used the same approach to estimate mtDNA abundance as the average mtDNA read depth normalized by the BRD. Homology between nuclear and mitochondrial ribosomal genes did not bias read depth for either the rDNA dosage or mtDNA abundance estimates, as none of the reads that mapped to the rDNA locus also mapped to the mitochondrion genome. The length of the targeted sequence (rDNA component and mtDNA genome) does not influence the estimates of read depth. Robustness of rDNA read mapping CN and dosage estimations are sensitive to read mapping. Sequence similarity between rDNA components could potentially confound read depth coverage and thus rDNA dosage quantification. We assessed sequence similarity between rDNA components by BLASTing each rDNA component against all other rDNA components ( E -value <1 × 10 −6 ) [56] . We also assessed sequence homology by aligning all pairwise combinations of rDNA components using CLUSTALW (default settings) [62] . Furthermore, we tested whether rDNA reads mapped to multiple rDNA components, as such a phenomenon could confound rDNA sequence read depth values. Reads that mapped to each component were independently extracted using the ‘samtools view’ function. Reads for each rDNA component were then mapped against all other rDNA components using the ‘sensitive’ option in Bowtie2 v2.0.5 (ref. 57 ). Correction factor for estimating dosage of rDNA components We tested whether rDNA reads aberrantly mapped to alternative regions of the genome (potential rDNA pseudogenes). This effect could inflate rDNA read depth values and rDNA dosage estimates. To test this issue, extracted reads from each rDNA component were independently mapped against the reference GRCh37 (hg19) human genome using Bowtie2 v2.0.5 (ref. 57 ). The number of reads mapping to each chromosome and supercontig were calculated from the mapping output bam file using the samtools ‘idxstats’ function. For each sample, and each component, we applied a correction factor to our original estimates of rDNA dosage by multiplying each rDNA component dosage by the percentage of reads mapping to expected chromosomes or supercontigs (chromosomes 13, 14, 15, 21, 22 and supercontig GL000220.1). Validation of CN estimates To validate our method of CN quantification, we measured CN of 6 genes previously characterized in 80 overlapping individuals [16] . For the 80 samples, entire read sets were mapped against the CCL3L1 , TBC1D3F , MBD3L3 , USP17L6P , FAM157B and PRR20A genes using Bowtie2 v2.0.5 (ref. 57 ). As BRD was nearly identical between exons and introns, we used the entire gene, from start codon to stop codon (including introns), for mapping. CN for each gene was calculated as described for the rDNA dosage quantification. For each gene, our results were plotted against results from Sudmant et al . [16] Linear regression analysis was used to assess the correlation of CN quantification between studies. Population structure and differentiation of rDNA dosage CEU and YRI display relatively small levels of population differentiation relative to other human population pairs [63] . It is also beneficial to our purposes that there is no evidence for population stratification within either CEU or YRI populations [63] , [64] . To further examine population differentiation specifically in rDNA dosage between CEU and YRI populations, we calculated V ST values for each rDNA component [60] . V ST , analogous to F ST , compares the variance in CNV within and between populations. V ST was calculated as ( V T – V S )/ V T , where V T is the variance in Log 2 ratios among all unrelated individuals and V S is the population size-weighted average variance within each population ( Fig. 4a ). In addition, we used PCA analysis to assess multivariate population differentiation in these loci. PCA was independently performed using the dosage estimates for the set of 45S rDNA components (18S, 5.8S and 28S), and the set of 45S components and the estimates of mtDNA abundance ( Fig. 4d,e ). Genome-wide association of rDNA dosage on GE Normalized mapped read results were obtained from the ReCount database ( http://bowtie-bio.sourceforge.net/recount/ ) [34] from two previous RNA-seq studies of lymphoblastoid cell lines [24] , [25] for 97 individuals with matched rDNA CN measurements (29 female CEU, 25 male CEU, 31 female YRI and 12 male YRI). For each sample, GE was measured as: We constrained our analysis to genes that were expressed in at least 50 samples, resulting in 7,841 genes with high-quality estimates of expression. Pearson’s product–moment correlation coefficient ( r ) was used to measure the association between rDNA CN and GE. Correlations were calculated for each rDNA component independently (18S, 5.8S and 28S). We combined the probabilities of the 18S, 5.8S and 28S rRNA genes using Fisher’s combined probability method [65] . The 18S, 5.8S and 28S rRNA genes are encoded within the same locus, their dosage levels were highly correlated ( Figs 1 and 2 ) and they share extensive overlap between significantly correlated genes ( Fig. 5a,b ). The relationship between mtDNA abundance and GE was estimated in the same manner. Finally, mixed effect linear models were used in the eQTL analyses. To test whether significantly correlated genes were represented disproportionately in particular chromosomes, we compared the proportion of observed and expected genes present on each chromosome assuming no chromosomal bias using a χ 2 goodness-of-fit test. To test whether significantly positively and negatively correlated genes were unevenly represented, we compared the observed frequencies to the expected frequencies assuming an equal distribution of correlation types. This hypothesis was tested using a χ 2 goodness-of-fit test. Finally, we tested whether the number of overlapping rDNA and mtDNA correlated genes were more abundant than expected by chance using a χ 2 goodness-of-fit test. The number of observed and expected overlapping genes and background genes were compared. The expected number of overlapping genes were calculated as total number of analysed genes × relative frequency of mtDNA significantly correlated genes × relative frequency of rDNA significantly correlated genes. Expected background genes were calculated as total number of analysed genes−expected number of overlapping genes. PCA analysis of expression estimates To account for factors that might influence global patterns of GE, we performed PCA analysis on the sample correlation matrix independently for each population. The first three principal components accounted for >95% of the variance in both CEU and YRI populations. We have computed the residuals from the regression between the first three principal components and each of the original estimates of expression values. These residuals were used as input for the eQTL analysis. The stability of the eQTL results between the original normalized expression estimates and the PC residuals were investigated in two ways. First, we compared the estimates of association in both analyses (that is, the stability of the Pearson correlations). Second, we carefully inspected the stability of functionally coherent gene sets. Overall, the analysis showed strong concordance between the associations estimated directly with normalized expression values or estimated on the residuals after removal of the first three principal components (18S: r =0.72, 5.8S: r =0.80 and 28S: r =0.80; for all comparisons, P <1 × 10 −300 ). Principal components were estimated and removed separately for each population. Population effects were estimated with linear models. GO enrichment of gene sets GO enrichment analysis was performed on subsets of genes using the GOrilla Gene Ontology enRIchment anaLysis and visuaLizAtion tool [66] . For this analysis, GO enrichment was performed on the target set of genes compared with the background set of genes (7,841 analysed genes−target set of genes). Enrichment was independently assessed against the Biological Processes, Molecular Function and Cellular Component ontologies implementing a P-value threshold 0.001. How to cite this article: Gibbons, J. G. et al . Ribosomal DNA copy number is coupled with gene expression variation and mitochondrial abundance in humans. Nat. Commun. 5:4850 doi: 10.1038/ncomms5850 (2014).